LaAlO3stoichiometry is key to electron liquid formation at LaAlO3/SrTiO3interfaces Emergent phenomena, including superconductivity and magnetism, found in the two-dimensional electron liquid (2-DEL) at the interface between the insulators lanthanum aluminate (LaAlO 3 ) and strontium titanate (SrTiO 3 ) distinguish this rich system from conventional 2D electron gases at compound semiconductor interfaces. The origin of this 2-DEL, however, is highly debated, with focus on the role of defects in the SrTiO 3 , while the LaAlO 3 has been assumed perfect. Here we demonstrate, through experiments and first-principle calculations, that the cation stoichiometry of the nominal LaAlO 3 layer is key to 2-DEL formation: only Al-rich LaAlO 3 results in a 2-DEL. Although extrinsic defects, including oxygen deficiency, are known to render LaAlO 3 /SrTiO 3 samples conducting, our results show that in the absence of such extrinsic defects an interface 2-DEL can form. Its origin is consistent with an intrinsic electronic reconstruction occurring to counteract a polarization catastrophe. This work provides insight for identifying other interfaces where emergent behaviours await discovery. The intriguing discovery of a two-dimensional electron liquid (2-DEL) [1] , [2] , [3] at the interface between two simple band insulators, lanthanum aluminate (LaAlO 3 ) and strontium titanate (SrTiO 3 ), and the subsequent observation of collective ground states, including superconductivity [4] , [5] , magnetism [6] , [7] and an unexpected coexistence of superconductivity and magnetism [8] , [9] , [10] , has fueled exciting research on the interactions between the confined electrons and their spin, orbital degrees of freedom [11] , [12] , [13] . The origin of this 2-DEL has been attributed to a “polar catastrophe”, an intrinsic electronic reconstruction [1] , [14] , [15] , [16] , [17] , [18] , which acts to remove the diverging electric potential caused by the atomic layer arrangement at the interface—(SrO) 0 -(TiO 2 ) 0 -(LaO) +1 -(AlO 2 ) −1 . This hypothesis for the origin of the observed interfacial conductivity has been questioned and there has been much debate as to the role of defects on the conductivity of this system [19] , [20] , [21] , [22] , [23] . Even though a growing number of experiments have provided evidence supporting the polar catastrophe mechanism [24] , [25] , the relatively high-energy and far-from-equilibrium growth conditions involved in pulsed-laser deposition (PLD), which has been at the forefront of the aforementioned discoveries, has raised concerns about defect-driven conductivity at the interface [22] , [23] . As the effect of the LaAlO 3 composition on interfacial conductivity has not been studied [26] , we study that here on samples mostly grown by molecular-beam epitaxy (MBE). Our experiments not only eliminate suggested extrinsic defect mechanisms as the origin of the interface conductivity, but show an unexpected dependence on the cation stoichiometry of the LaAlO 3 film for the formation of an interfacial 2-DEL. Our results reveal that a La/Al ratio ≤0.97±0.03 is a necessary condition for obtaining a 2-DEL at the interface between LaAlO 3 and TiO 2 -terminated (001) SrTiO 3 . Our studies further show that this result is also consistent with samples grown by PLD [2] . Mosaic growth experiment To investigate the effect of LaAlO 3 stoichiometry on the 2-DEL, as well as the role of substrate preparation, growth conditions and intermixing at the interface, we grew simultaneously on a mosaic of substrates mounted on a sample holder ( Fig. 1a ), with a monotonic variation in the La/Al ratio across the LaAlO 3 film achieved from the placement of the sources in the MBE system (see Methods). These 16 substrates were obtained from cutting four, 10 mm × 10 mm, TiO 2 -terminated (001) SrTiO 3 substrates (labelled 1, 2, 3 and 4) each into four 5 mm × 5 mm pieces (labelled A, B, C and D). The mosaic was formed by mounting pieces from different substrates next to each other. With lanthanum and aluminum fluxes calibrated to within a few per cent, the gradient in the La/Al ratio ensured that at some position on the mosaic, stoichiometric LaAlO 3 was deposited. It also provided a means to explore the effect of small composition variations in La (1− δ ) Al (1+ δ ) O 3 on the resulting electronic properties at the interface. This growth experiment was repeated three times. In each growth, the position on the mosaic where stoichiometric LaAlO 3 was expected was moved by adjusting the shutter-open times of lanthanum and aluminum for the growth of each monolayer based on the in-situ flux calibration that preceded the mosaic growth (see Supplementary Note 1 ). Immediately following each growth, a companion calibration sample was also grown on which ex-situ Rutherford backscattering spectrometry (RBS) measurements were performed to determine the position of stoichiometric LaAlO 3 (see below). This position is indicated for each mosaic in Fig. 1a by a white circle. Moving to the left of the white circle increases the La/Al ratio, given by (1− δ )/(1+ δ ), beyond 1, whereas moving to the right decreases the La/Al ratio below 1. 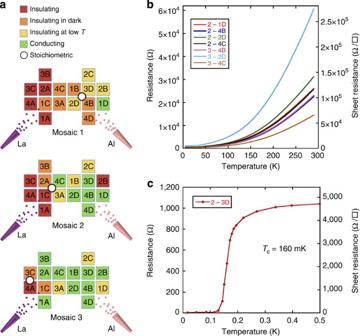Figure 1: Flux gradients and interfacial conductivity of mosaic samples. (a) Mosaic arrangement of substrates for each growth. The location of lanthanum and aluminum effusion cells relative to the mosaic of substrates is also indicated. The La/Al ratio decreases on moving from left to right across each mosaic. The position of stoichiometric LaAlO3, determined byex situRBS measurements for each mosaic growth, is shown by a white circle. Samples with a conducting interface are shown in green and are only found to the right of the white circle in each mosaic. (b) Temperature dependence of resistance of the 2-DEL is plotted for a representative set of conducting samples from the mosaic growths. The samples are labelled with the mosaic number followed by substrate number—for example, 2–1D indicates mosaic 2, piece D of substrate 1. (c) A representative low-temperature resistance versus temperature plot shows the 2-DEL is superconducting. The scaling between resistance and sheet resistance is approximate. Figure 1: Flux gradients and interfacial conductivity of mosaic samples. ( a ) Mosaic arrangement of substrates for each growth. The location of lanthanum and aluminum effusion cells relative to the mosaic of substrates is also indicated. The La/Al ratio decreases on moving from left to right across each mosaic. The position of stoichiometric LaAlO 3 , determined by ex situ RBS measurements for each mosaic growth, is shown by a white circle. Samples with a conducting interface are shown in green and are only found to the right of the white circle in each mosaic. ( b ) Temperature dependence of resistance of the 2-DEL is plotted for a representative set of conducting samples from the mosaic growths. The samples are labelled with the mosaic number followed by substrate number—for example, 2–1D indicates mosaic 2, piece D of substrate 1. ( c ) A representative low-temperature resistance versus temperature plot shows the 2-DEL is superconducting. The scaling between resistance and sheet resistance is approximate. Full size image The interfacial electronic properties of each mosaic sample were probed with contacts made to the interfaces patterned using photolithography (see Methods for patterning details). In all three mosaic experiments, conducting interfaces (indicated in green in Fig. 1a ) were found only in samples that were mounted to the right of the white circle, where La/Al <1, regardless of the substrate from which the samples originated. Figure 1b shows the temperature dependence of the resistance of many of the conducting interfaces obtained from the mosaic experiments. A residual resistivity ratio (resistance at 290 K/resistance at 4 K) of the order of 50 is observed in these conducting samples and an average sheet-carrier density of ~1.5 × 10 13 cm −2 is found using low-temperature Hall measurements. Most of these conducting samples are also found to be superconducting, with superconducting critical temperatures between 150 and 250 mK. A representative superconducting transition is shown in Fig. 1c . The conductivity and superconductivity observed in these samples are comparable to those reported in PLD-grown samples [2] , [4] , [5] . Evidence eliminating extrinsic mechanisms of conduction This mosaic growth experiment eliminates four of the proposed extrinsic causes of conductivity in LaAlO 3 /(001) SrTiO 3 samples: (1) oxygen vacancies in the SrTiO 3 due to insufficiently oxidizing conditions during growth or during an oxygen annealing step after growth [19] , [20] , [21] , [27] , (2) high concentrations of oxygen vacancies in the surface region of etched and annealed SrTiO 3 substrates prepared by the preferred substrate termination etch for (001) SrTiO 3 (ref. 28 , 3) bombardment of the SrTiO 3 by energetic species during growth leading to oxygen vacancies [29] and (4) chemical mixing of lanthanum from the LaAlO 3 with the SrTiO 3 to make La-doped SrTiO 3 (ref. 30 ), a known conductor and superconductor. LaAlO 3 films were grown on all of the SrTiO 3 pieces (cut from four different substrates) at the same time by MBE. If the growth conditions were insufficient to oxidize one of them, the other pieces cut from the same substrate need also be conducting, thus eliminating hypothesis 1. Similarly, hypothesis 2 can be eliminated, as all SrTiO 3 pieces were prepared using the same TiO 2 termination procedure for (001) SrTiO 3 (ref. 31 ), but a 2-DEL was found only in some pieces of each substrate. In contrast to PLD growth, where conditions may exist for high-energy species to bombard the growing film and produce various types of extrinsic defects [32] , [33] , [34] , MBE affords a gentle means of film growth utilizing only thermal beams of neutral species, including the purified ozone beam used as the oxidant, with energies <1 eV. This eliminates hypothesis 3. Finally, LaAlO 3 is in contact with SrTiO 3 on all of the simultaneously grown wafers, so if intermixing (hypothesis 4) is relevant, the intermixing is only active in samples containing certain compositions. All the three mosaic experiments that cover an even larger composition space show that La-rich compositions—where the most interdiffusion might be expected—are, in fact, not conducting. The interfaces of both conducting and non-conducting samples from the same mosaic growth were chemically mapped using cross-sectional scanning transmission electron microscopy with electron energy loss spectroscopy (STEM-EELS). The high-angle annular dark-field STEM images in Fig. 2 show LaAlO 3 /SrTiO 3 interfaces of representative insulating and conducting interfaces near the ends of the stoichiometry range explored. EELS spectroscopic imaging revealed a small amount of lanthanum interdiffusion (<0.1%) into the substrate for both conducting and insulating samples ( Fig. 2c ). Critically, the lanthanum interdiffusion was not correlated to the La (1− δ ) Al (1+ δ ) O 3 stoichiometry or the conductivity, ruling out hypothesis 4. Fine structure analysis of the O – K edge showed a distinct interface component with the same concentration and spatial extent for both conducting and insulating samples ( Supplementary Fig. S2 ). Changes in the titanium valence were below the sensitivity threshold of the microscope ( Supplementary Fig. S3 ). Further, from measurements made on plan-view samples, we find the density and spacing of interfacial dislocations at the SrTiO 3 /LaAlO 3 interface to be comparable (~38±3 nm versus 43±3 nm between dislocations for conducting and insulating samples 2–4B and 2–4A, respectively). 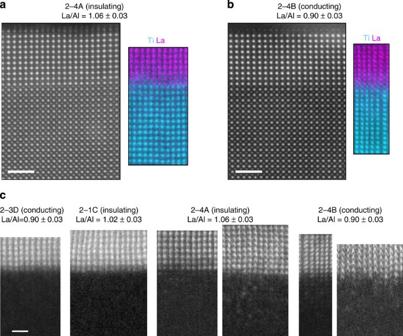Figure 2: High-angle annular dark-field STEM images and EELS spectroscopic maps. (a) An insulating sample 2–4A (with La/Al=1.06±0.03). Scale bar, 2 nm. (b) A conducting sample 2–4B (with La/Al=0.90±0.03). Scale bar, 2 nm. The high-angle annular dark-field (HAADF) STEM images show that both regions have coherent interfaces. The EELS spectroscopic images map the concentration of lanthanum in magenta and titanium in turquoise; both samples show a small amount of interdiffusion at the interface. (c) EELS maps of lanthanum for several samples from Mosaic 2 are ordered from left to right by the increasing degree of interdiffusion. Scale bar, 1 nm. No correlation between lanthanum interdiffusion and interface conductivity is observed. Slight distortions in the maps are due to drift and charging during acquisition. Figure 2: High-angle annular dark-field STEM images and EELS spectroscopic maps. ( a ) An insulating sample 2–4A (with La/Al=1.06±0.03). Scale bar, 2 nm. ( b ) A conducting sample 2–4B (with La/Al=0.90±0.03). Scale bar, 2 nm. The high-angle annular dark-field (HAADF) STEM images show that both regions have coherent interfaces. The EELS spectroscopic images map the concentration of lanthanum in magenta and titanium in turquoise; both samples show a small amount of interdiffusion at the interface. ( c ) EELS maps of lanthanum for several samples from Mosaic 2 are ordered from left to right by the increasing degree of interdiffusion. Scale bar, 1 nm. No correlation between lanthanum interdiffusion and interface conductivity is observed. Slight distortions in the maps are due to drift and charging during acquisition. Full size image Effect of La (1− δ ) Al (1+ δ ) O 3 stoichiometry on 2-DEL formation To more accurately and quantitatively determine the effect of LaAlO 3 stoichiometry on 2-DEL formation, we grew on (001) SrTiO 3 crystalline substrates that were ~25 mm long (see Methods). Immediately following the growth of a calibration sample (see Supplementary Note 1 ), three such long samples were grown back-to-back. The La/Al ratio at the centre of each sample was varied by adjusting the shutter-open times of lanthanum and aluminum sources for the growth of each monolayer. Immediately following the growth of the three samples, a companion RBS calibration sample was also grown. The structure of the RBS calibration samples and their analysis is described in the next section. 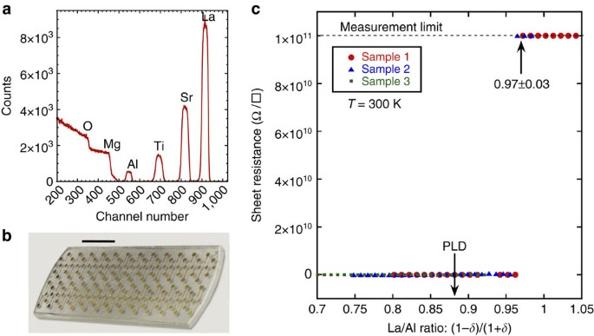Figure 3: Interfacial conductivity and its dependence on La/Al ratio of La(1−δ)Al(1+δ)O3films. (a) Representative RBS spectrum from a companion sample. Well-separated peaks obtained, especially for aluminum, due to the structure of the companion RBS samples, enabled accurate calibration measurements by peak integration. (b) Patterning of an ~25-mm-long La(1−δ)Al(1+δ)O3/(001) SrTiO3sample allowed local four-point transport measurements to be made at 1-mm intervals. Scale bar, 5 mm. Note that the shadows of the Ti/Au contacts are visible through the transparent sample. (c) Room temperature sheet resistance of La(1−δ)Al(1+δ)O3/(001) SrTiO3interfaces obtained by local four-point resistance measurements is plotted as a function of the La/Al ratio determined by RBS measurements. A sharp jump in sheet resistance is observed at La/Al=0.97±0.03, consistently in all three samples. See text for error analysis and seeSupplementary Fig. S4for resistance of conducting devices. An arrow indicates the stoichiometry of a PLD-grown companion sample similar to the samples studied in ref.2. Figure 3a shows a representative RBS spectrum from a companion calibration sample. The La/Al ratio at the centre of each long sample was determined from peak integration of the RBS spectrum of the companion calibration sample. The relative spatial variation of the La/Al ratio was also determined to better than ±3% accuracy through separate RBS experiments ( Fig. 4 ). From these RBS measurements, the absolute spatial variation of the La/Al ratio of the three long La (1− δ ) Al (1+ δ ) O 3 /SrTiO 3 samples was determined. Figure 3: Interfacial conductivity and its dependence on La/Al ratio of La (1− δ ) Al (1+ δ ) O 3 films. ( a ) Representative RBS spectrum from a companion sample. Well-separated peaks obtained, especially for aluminum, due to the structure of the companion RBS samples, enabled accurate calibration measurements by peak integration. ( b ) Patterning of an ~25-mm-long La (1− δ ) Al (1+ δ ) O 3 /(001) SrTiO 3 sample allowed local four-point transport measurements to be made at 1-mm intervals. Scale bar, 5 mm. Note that the shadows of the Ti/Au contacts are visible through the transparent sample. ( c ) Room temperature sheet resistance of La (1− δ ) Al (1+ δ ) O 3 /(001) SrTiO 3 interfaces obtained by local four-point resistance measurements is plotted as a function of the La/Al ratio determined by RBS measurements. A sharp jump in sheet resistance is observed at La/Al=0.97±0.03, consistently in all three samples. See text for error analysis and see Supplementary Fig. S4 for resistance of conducting devices. An arrow indicates the stoichiometry of a PLD-grown companion sample similar to the samples studied in ref. 2 . 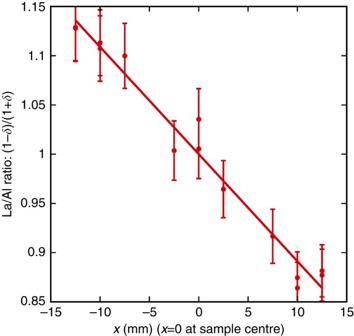Figure 4: Relative spatial variation of La/Al ratio. The relative variation in the La/Al ratio along the left-to-right (x) direction due to the placement of sources in the MBE system, obtained from multiple RBS measurements, is plotted. The error bars are based on the convolution of several sources of error, including RBS counting error and RBS measurement spot position error. The conservative estimate of each error source is used to find the convoluted error. Full size image Figure 4: Relative spatial variation of La/Al ratio. The relative variation in the La/Al ratio along the left-to-right ( x ) direction due to the placement of sources in the MBE system, obtained from multiple RBS measurements, is plotted. The error bars are based on the convolution of several sources of error, including RBS counting error and RBS measurement spot position error. The conservative estimate of each error source is used to find the convoluted error. Full size image The long La (1− δ ) Al (1+ δ ) O 3 /SrTiO 3 samples were patterned (see Methods) to enable four-point transport measurements every 1 mm along the ~25 mm length of the samples ( Fig. 3b ). This 1-mm spatial separation roughly corresponded to a 1% change in the La/Al ratio. Room-temperature resistance measurements made on these three samples are plotted as a function of the La/Al ratio ( Fig. 3c and Supplementary Fig. S4 ). Note that the three long samples are offset from each other in their span of the La/Al ratio. The transport data of all three samples are, however, consistent with a sharp insulator-to-metal transition that occurs at La/Al ratio, (1− δ )/(1+ δ )≤0.97±0.03. This transition is also consistent with the multiple experiments involving a mosaic spread of samples ( Fig. 1a ). The composition of a LaAlO 3 sample grown in the same PLD system and under similar growth conditions as the samples with conducting interfaces studied in ref. 2 was also measured. This RBS measurement yielded a spectrum similar to that shown in Fig. 3a . An arrow in Fig. 3c indicates the stoichiometry of the PLD-grown sample. This measurement further supports the result that La/Al≤0.97±0.03 is a necessary condition for obtaining a 2-DEL at La (1− δ ) Al (1+ δ ) O 3 /SrTiO 3 interfaces and suggests that this result is independent of the growth method used as long as the growth conditions do not promote extrinsic defects. The non-conducting interfaces reported in sputtered films that are found to be La-rich [35] is also consistent with our result (see Supplementary Note 2 ). Cation stoichiometry from RBS measurements The accuracy with which the cation stoichiometry can be predicted relies on the accuracy with which the RBS data can be extracted and how well the different peaks can be separated in the RBS spectrum. With aluminum being a light element, extracting accurate cation stoichiometry using RBS measurements for a film containing aluminum is inherently a very challenging process. This is because peaks of constituent elements of many substrates (for example, SrTiO 3 ) would bury the aluminum peak. Even if the LaAlO 3 film were grown on a silicon substrate for RBS measurements, the aluminum peak would be underneath the silicon peak, making it impossible to extract an accurate number density for aluminum in the sample. Similarly, if an MgO substrate was used for this purpose, the aluminum peak would be riding the shoulder of the magnesium peak, leading to the same problem. Thus, an important part of this experiment was the specially structured companion sample that was used for all RBS measurements. The companion sample was grown on a (001) MgO substrate on which an ~500-Å-thick buffer layer of SrTiO 3 was grown before growing the LaAlO 3 layer that was to be calibrated. The LaAlO 3 layer was also ~400 Å thick, to obtain a low statistical error, and was grown immediately following the device sample. The purpose of the intermediate SrTiO 3 film was to lower the energy of the α-particles, as they penetrated through the intermediate film before being scattered off the substrate. This moved the substrate magnesium peak to sufficiently lower energies such that the aluminum peak was clearly separated from the magnesium peak. From the RBS spectrum of the companion sample ( Fig. 3a ), by peak integration, an accurate measurement of the La/Al ratio at the centre of the device sample was determined. To obtain the spatial variation of the La/Al ratio across the La (1− δ ) Al (1+ δ ) O 3 films grown on the long (001) SrTiO 3 crystals, two separate RBS calibration samples were grown, where the calibration samples also spanned the spatial extent of the long SrTiO 3 crystals. These RBS calibration samples were structured similarly to the companion RBS samples. RBS data were measured as a function of the position on each of these two calibration growths. It should be noted that the spatial variation of the La/Al ratio, (1− δ )/(1+ δ ), is dependent only on the configuration of the MBE system when the same growth conditions are used. From the spatially resolved RBS measurements, it was observed that for our system the variation in the La/Al ratio was mostly along the left-to-right ( x ) direction. To obtain the relative spatial variation of the La/Al ratio, (1− δ )/(1+ δ ), along the x direction for any sample, the La/Al ratio at the centre of each of the calibration RBS samples was scaled to (1− δ )/(1+ δ )=1. This data ( Fig. 4 ), which provides the spatial variation of the La/Al ratio across a sample along the x direction, together with the data from the companion RBS sample that provides the absolute La/Al ratio at the centre of the device sample, makes it possible to accurately determine the La/Al ratio, (1− δ )/(1+ δ ) at any point of the long La (1− δ ) Al (1+ δ ) O 3 /(001) SrTiO 3 samples. The sheet resistance of each device of the three long samples is plotted in Fig. 3c and in Supplementary Fig. S4 as a function of the La/Al ratio, (1− δ )/(1+ δ ), obtained as discussed above. The error associated with the La/Al ratio is due to the convolution of four sources of error: RBS counting error (0.5–1.0%), spatial determination of the RBS measurement spot position (1.5–2%), drift in source fluxes between consecutive growths—from device sample to companion RBS sample (1–2%), and device position/placement (±1 mm) from the centre of the sample (1–1.2%). The estimated range for each error source is shown in parenthesis. This leads to a convoluted error in (1− δ )/(1+ δ ) of 2% (taking the lower estimates) or 3% (from the more conservative estimates). The conservative error estimate is reported for the La/Al ratio, (1− δ )/(1+ δ ). Density functional calculations The La (1− δ ) Al (1+ δ ) O 3 film accommodates different La/Al ratios by forming defects. We performed density functional calculations to determine the energetically favoured defects as a function of the La/Al ratio (see Supplementary Note 3 ). Supercells of bulk LaAlO 3 strained to the SrTiO 3 lattice constant were used. For La/Al ratios below 1, the excess aluminum substitutes for lanthanum. Each substitutional Al 3+ displaces from the ideal La 3+ position to bond with five oxygen ions ( Fig. 5a and Supplementary Fig. S12 ), resulting in a dipole moment but no net charge. For La/Al ratios above 1, the excess lanthanum cannot substitute for aluminum, and Al 2 O 3 -vacancy complexes form as shown in Fig. 5d . Larger Al 2 O 3 -vacancy complexes (see Supplementary Fig. S5 ) relieve more strain in the films and have lower energy. 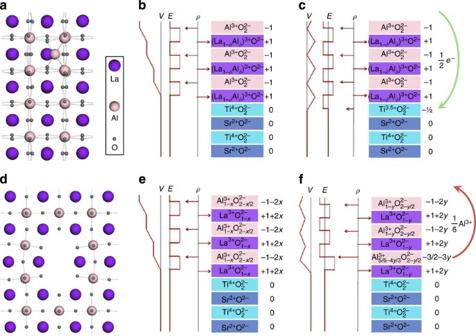Figure 5: Lowest energy structures and illustrations of the polar catastrophe. (a) In Al-rich films, aluminum substitutes for lanthanum and shifts off the cuboctahedron centre. The lowest-energy structure is shown as viewed along the [100] direction. (b) The alternating charges (ρ) of the (001) planes in Al-rich La(1−δ)Al(1+δ)O3and the charge neutral (001) planes in SrTiO3generates a positive average electric field (E) and a diverging potential (V). Note:ρ/ε=·E=−2V. The substitution of Al3+for La3+does not modify the alternating polarity from that of a stoichiometric LaAlO3film. (c) In thick Al-rich films, the system reconstructs electronically, transferring half an electron per unit cell from the surface to the interface. (d) In La-rich films, Al2O3-vacancy complexes form, which are periodic in the [001] direction. The smallest Al2O3-vacancy complex is shown as viewed along the [001] direction. (e) The extended Al2O3-vacancy complexes in the unreconstructed La-rich films also remove oxygen from the nominal (LaO)+layers. The aluminum deficiency is given byx=−2δ/(1−δ). A diverging potential results in the unreconstructed films from the alternately charged (001) planes of La(1−δ)Al(1+δ)O3. (f) In thick La-rich films, extra aluminum vacancies can move to the interface through the Al2O3-vacancy complexes to screen the diverging potential. The aluminum deficiencyynow depends on the stoichiometry (δ) and the film thickness. Figure 5: Lowest energy structures and illustrations of the polar catastrophe. ( a ) In Al-rich films, aluminum substitutes for lanthanum and shifts off the cuboctahedron centre. The lowest-energy structure is shown as viewed along the [100] direction. ( b ) The alternating charges ( ρ ) of the (001) planes in Al-rich La (1− δ ) Al (1+ δ ) O 3 and the charge neutral (001) planes in SrTiO 3 generates a positive average electric field ( E ) and a diverging potential ( V ). Note: ρ / ε = · E =− 2 V . The substitution of Al 3+ for La 3+ does not modify the alternating polarity from that of a stoichiometric LaAlO 3 film. ( c ) In thick Al-rich films, the system reconstructs electronically, transferring half an electron per unit cell from the surface to the interface. ( d ) In La-rich films, Al 2 O 3 -vacancy complexes form, which are periodic in the [001] direction. The smallest Al 2 O 3 -vacancy complex is shown as viewed along the [001] direction. ( e ) The extended Al 2 O 3 -vacancy complexes in the unreconstructed La-rich films also remove oxygen from the nominal (LaO) + layers. The aluminum deficiency is given by x =−2 δ /(1− δ ). A diverging potential results in the unreconstructed films from the alternately charged (001) planes of La (1− δ ) Al (1+ δ ) O 3 . ( f ) In thick La-rich films, extra aluminum vacancies can move to the interface through the Al 2 O 3 -vacancy complexes to screen the diverging potential. The aluminum deficiency y now depends on the stoichiometry ( δ ) and the film thickness. Full size image The large electric field density in ideal films of LaAlO 3 on TiO 2 -terminated (001) SrTiO 3 has an energy cost. Negative charges at the interface screen this field, and indeed density functional calculations simulating thick films of LaAlO 3 on SrTiO 3 show the interface is unstable to the formation of cation vacancies. For La/Al>1, the Al 2 O 3 -vacancy complexes provide conduits for cations to move from the interface. With the positive charge associated with the cations that have moved away from the interface missing, the field is screened and the interface remains insulating (see, for example, Fig. 5e,f ). In contrast, for La/Al≤1, the aluminum substitutional defects block migration of cations from the interface to form vacancies, resulting in electronic charge to transfer from the surface to the interface and form a 2-DEL to avoid a polar catastrophe ( Fig. 5b,c ). It is likely that a surface reconstruction accompanies the electronic charge transfer to the interface—density functional calculations have shown that oxygen vacancies on the surface have negative formation energy at LaAlO 3 thicknesses greater than 3 unit cells [36] . There will be local fluctuations, however, in the stoichiometry of the grown films. For example, films grown on stoichiometry will have Al-rich regions and La-rich regions. We suspect that a percolating network of these local stoichiometry variations shifts the critical La/Al ratio to the smaller value (0.97±0.03) seen in the experiments. Cation composition mapping using STEM-EELS To assess the above theory predicting different types of defects in films with La/Al>1 from those with La/Al<1, we utilized atomic-resolution STEM-EELS to determine layer-to-layer variations in cation occupancy along the [001] growth direction. Spectroscopic images of lanthanum and strontium, as well as of aluminum and titanium, were collected simultaneously to map the total concentration of cations residing on the A -site and B -site sublattices, respectively (see Supplementary Note 4 for details). In the conducting, Al-rich samples, aluminum and titanium were found to completely occupy the B -site sublattice, as shown in Fig. 6b . In contrast, the insulating, La-rich samples show a local accumulation of cation vacancies on the B -site sublattice at the interface ( Fig. 6d ). 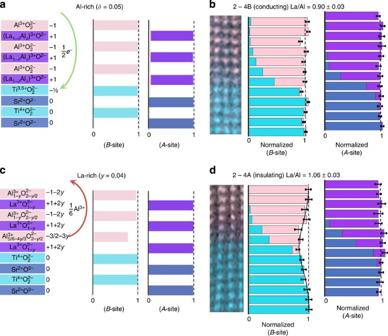Figure 6: Cation concentrations from theory and atomic-resolution STEM-EELS. (a)A-site andB-site cation occupancies found, from theory, for Al-rich structure shown inFig. 5cwithδ=0.05. Although aluminum substitutional defects are included as part of theA-site occupancy, they are shifted off centre as shown inFig. 5a. (b) A representative STEM-EELS spectroscopic image of aluminum (pink) and titanium (turquoise) from the conducting wafer 2–4B shown inFig. 2b. The normalized aggregate concentration of titanium and aluminum occupying theB-site sublattice does not show any systematic variation from layer to layer along the [001] direction. Similarly, the aggregate occupancy of lanthanum and strontium at theA-site shows no variation along the [001] direction. (c)A-site andB-site cation occupancies found, from theory, for La-rich structure shown inFig. 5fwithy=0.04. Note the cation deficiency in theB-site at the interface. (d) A representative STEM-EELS spectroscopic image of aluminum (pink) and titanium (turquoise) from the insulating wafer 2–4A shown inFig. 2a. In contrast to the map shown inb, there is a dip in the normalizedB-site occupancy at the interface, indicating a local accumulation ofB-site vacancies, whereas theA-site occupancy shows no detectable variation along the [001] direction. Figure 6b,d also shows that neither interface shows a corresponding local dip in the cation concentration on the A -site sublattice. The experimentally observed cation vacancies in the B -site sublattice at the interface of La-rich samples ( Fig. 6d ) are significant for understanding the charge balance at the interface. Density functional calculations show that these cation vacancies alleviate the polar catastrophe ( Fig. 5f and Fig. 6c ) without the transfer of electronic charge to the interface to form a 2-DEL. Figure 6: Cation concentrations from theory and atomic-resolution STEM-EELS. ( a ) A -site and B -site cation occupancies found, from theory, for Al-rich structure shown in Fig. 5c with δ =0.05. Although aluminum substitutional defects are included as part of the A -site occupancy, they are shifted off centre as shown in Fig. 5a . ( b ) A representative STEM-EELS spectroscopic image of aluminum (pink) and titanium (turquoise) from the conducting wafer 2–4B shown in Fig. 2b . The normalized aggregate concentration of titanium and aluminum occupying the B -site sublattice does not show any systematic variation from layer to layer along the [001] direction. Similarly, the aggregate occupancy of lanthanum and strontium at the A -site shows no variation along the [001] direction. ( c ) A -site and B -site cation occupancies found, from theory, for La-rich structure shown in Fig. 5f with y =0.04. Note the cation deficiency in the B -site at the interface. ( d ) A representative STEM-EELS spectroscopic image of aluminum (pink) and titanium (turquoise) from the insulating wafer 2–4A shown in Fig. 2a . In contrast to the map shown in b , there is a dip in the normalized B -site occupancy at the interface, indicating a local accumulation of B -site vacancies, whereas the A -site occupancy shows no detectable variation along the [001] direction. Full size image It is well known that extrinsic defects can lead to conductivity in SrTiO 3 and in LaAlO 3 /(001) SrTiO 3 samples. The question has been whether there could be an intrinsic mechanism, such as the polar catastrophe, that could lead to conductivity at the interface between the two band insulators. Our uniquely implemented growth experiments involving over 50 samples together with careful stoichiometry measurements have answered this question by comparing conductive and insulating interfaces grown simultaneously, even on the same substrate. Minor differences in the stoichiometry of the La (1− δ ) Al (1+ δ ) O 3 films correlate to the abrupt change from conducting to insulating samples at a critical La/Al ratio of 0.97±0.03. This result, consistent with the critical thickness found [2] , [25] in samples grown over a large span of oxygen concentrations, further supports that oxygen vacancies cannot be the driver of conductivity (also see Supplementary Note 5 ). The ability to compare insulating and conducting interfaces in our sample set has enabled us to assess which characteristics correlate with conductive interfaces and which do not. None of the proposed extrinsic mechanisms—(1) oxygen vacancies in the SrTiO 3 due to insufficiently oxidizing conditions [19] , [20] , [21] , [27] , (2) high concentrations of oxygen vacancies in the surface region of etched and annealed SrTiO 3 substrates [28] , (3) bombardment of the SrTiO 3 by energetic species during growth [29] or (4) chemical mixing of lanthanum from the LaAlO 3 with the SrTiO 3 (ref. 30 )—can explain the sharp transition from conducting to insulating interfaces in our sample set. This is not to say that the above mechanisms cannot lead to conductive samples, they easily can; it is only to say that in our sample set, some other mechanism is at work to make the Al-rich interfaces conductive. Having ruled out all proposed extrinsic defect mechanisms for the observed 2-DEL in our samples, we have considered how it is that a small change in the La (1− δ ) Al (1+ δ ) O 3 film composition could lead to the abrupt change in interface conductivity. Our direct spectroscopic observation of the accumulation of cation vacancies near the interface in La-rich samples and its correlation with insulating interfaces introduces a new factor relevant to 2-DEL formation—cation vacancies. By measuring the B -site vacancy content across both conductive and insulating LaAlO 3 /SrTiO 3 interfaces (grown simultaneously, side-by-side on pieces of the same substrate), we find the insulating interfaces consistently show B -site vacancies, whereas the conducting interfaces do not. Our observations, supported by first-principle calculations, point to different pathways for compensating the polar discontinuity at the heterointerface: in La-rich samples, cation vacancies form at the interface to avoid the polarization catastrophe, which lead to insulating interfaces, whereas in Al-rich samples the diffusion of cations away from the interface is blocked and an electronic reconstruction occurs to counteract the polarization catastrophe, giving rise to a 2-DEL. Our experiments thus show that a 2-DEL can form at the interface between La (1− δ ) Al (1+δ) O 3 and TiO 2 -terminated (001) SrTiO 3 substrates in the absence of any of the previously proposed extrinsic defect mechanisms that are known to cause conductivity in bulk SrTiO 3 . Further, our results point to the polar catastrophe model; in insulating (La-rich) samples, the predicted and observed local accumulation of cation vacancies on the B -site in the vicinity of the interface acts to remove the diverging potential, whereas this is accomplished in conducting (Al-rich) samples by an electronic reconstruction that forms a 2-DEL. The different responses operative in the oxide heterostructures to defects as deduced by our work on La-rich and Al-rich films grown on TiO 2 -terminated (001) SrTiO 3 show that controlling the composition of the overlying La (1− δ ) Al (1+ δ ) O 3 is key to 2-DEL formation. This result likely extends to other interfaces with mismatched polarity and lattice strain [25] , [37] , [38] , [39] , [40] in which a polar discontinuity governs the interface electronic properties. The delicate balance between cation stoichiometry we find to be key is, however, absent in the binary oxide γ-Al 2 O 3 films grown on (001) SrTiO 3 (ref. 40 ). At first sight the interface conductivity in this system does not seem surprising, because it was reported to arise from a conventional, growth-induced reduction of a SrTiO 3 surface layer rather than from a polar catastrophe [40] . But, Sawatzky (2013, personal communication) has pointed out that when the cation site occupancy of the γ-Al 2 O 3 structure is taken into account, the conductivity at the γ-Al 2 O 3 /SrTiO 3 interface is found to completely match the polar catastrophe mechanism, because γ-Al 2 O 3 consists of alternating charged layers along the [001] growth direction. Thus, the need to evaluate competing responses, such as ionic motions and electronic reconstructions that avert a polar catastrophe, is important for the physics of 2-DELs and the collective ground states that occur not only at perovskite-based interfaces but also at buried oxide interfaces based on non-perovskite systems. Elemental flux gradients To explore whether the conductivity at the LaAlO 3 –SrTiO 3 interface is generated by PLD-specific defects as suggested [22] , [23] , [29] , we grew LaAlO 3 –SrTiO 3 interfaces by MBE. In contrast to PLD where a multicomponent target and molecular oxygen are typically used, the oxide heterostructures grown via MBE utilized separate elemental sources of the constituents, including distilled ozone as the oxidant. The geometry between the effusion cells and the substrate in our MBE experiments was selected to produce flux gradients of lanthanum and aluminum in nearly opposite directions across the sample. As the sample was not rotated during growth, the La/Al ratio across the La (1− δ ) Al (1+ δ ) O 3 film could be monotonically varied, while ensuring that at some position on the sample stoichiometric LaAlO 3 was deposited, provided the lanthanum and aluminum fluxes were calibrated to within a few per cent (see Supplementary Note 1 for in-situ flux calibration details). La (1− δ ) Al (1+ δ ) O 3 film growth All SrTiO 3 substrates were prepared to have a TiO 2 -terminated surface [31] . The LaAlO 3 films were grown in a background partial pressure of distilled ozone of 1 × 10 −6 torr at a substrate temperature of 680 °C in a Veeco 930 MBE. The LaAlO 3 films were grown starting with a LaO monolayer followed by an AlO 2 monolayer. This monolayer sequence was repeated to obtain an eight-unit-cell-thick film of LaAlO 3 . The growth rate was kept at ~60 s per monolayer. After growth, the samples were cooled to below 200 °C while maintaining the same background partial pressure of distilled ozone. SrTiO 3 substrates, when subjected to these same growth conditions except for the deposition of the La (1-δ) Al (1+δ) O 3 , did not show any signs of conductivity (see Supplementary Note 5 ). Patterning and processing for measurements Electrical contacts were patterned utilizing photolithography to contact the interface 2-DEL by ion milling the contact areas with argon, followed by titanium and gold deposition [2] . Contacts to the mosaic samples were made in a square geometry around the edge of the samples. For the long samples, a mask was used to enable local four-point measurements spaced 1 mm apart as shown in Fig. 3b . High-angle annular dark-field STEM images and EELS spectroscopic images were recorded from cross-sectional TEM specimens using a 100 keV NION UltraSTEM. How to cite this article: Warusawithana, M. P. et al . LaAlO 3 stoichiometry is key to electron liquid formation at LaAlO 3 /SrTiO 3 interfaces. Nat. Commun. 4:2351 doi: 10.1038/ncomms3351 (2013).